Automated monitoring and quantitative analysis of feeding behaviour inDrosophila Food ingestion is one of the defining behaviours of all animals, but its quantification and analysis remain challenging. This is especially the case for feeding behaviour in small, genetically tractable animals such as Drosophila melanogaster . Here, we present a method based on capacitive measurements, which allows the detailed, automated and high-throughput quantification of feeding behaviour. Using this method, we were able to measure the volume ingested in single sips of an individual, and monitor the absorption of food with high temporal resolution. We demonstrate that flies ingest food by rhythmically extending their proboscis with a frequency that is not modulated by the internal state of the animal. Instead, hunger and satiety homeostatically modulate the microstructure of feeding. These results highlight similarities of food intake regulation between insects, rodents, and humans, pointing to a common strategy in how the nervous systems of different animals control food intake. Feeding is an essential component of an animal’s behavioural repertoire and forms a mechanistic link between physiology and behaviour [1] . Fruit flies ( Drosophila melanogaster) have emerged as a powerful model to study the neuronal and molecular mechanisms underlying feeding behaviour [2] , [3] , [4] , [5] , [6] , [7] , [8] , but it remains challenging to quantify feeding in these tiny insects, due to the minute quantities of food they ingest. Most current methods rely either on manual scoring of proboscis extensions [9] , post hoc quantification of the ingested food using colourants [10] or radioactive substances [11] or measurement of the volumetric change of food ingested from a capillary [5] . Although widely employed, these methods have several limitations. For example, they do not provide the sensitivity to monitor food intake by individual animals over time, they force the animals to feed from specialized devices in restricted positions, or they require the addition of dyes or radioactive labels. These drawbacks limit the feasibility of high throughput, unbiased studies of feeding as well as the identification of important behavioural parameters controlling food selection and intake. In rodents [12] , [13] , humans [14] and insects [15] , the microstructure of ‘meals’ has been very valuable in providing insights into how hunger and satiation regulate homeostasis. Advancing our understanding of homeostasis in flies would benefit from a method that provides sufficient sensitivity and temporal resolution to quantify each ingestion event. In recent years, several automated and quantitative approaches have emerged to monitor and analyse behaviour based on machine vision [16] , [17] . Because of the limitations of digital cameras, it is difficult to resolve the fine details of an animal’s physical interactions with small objects, such as morsels of food, especially if the system is optimized to track the animal over many body lengths. An alternative strategy for detecting fine-scale interactions between an animal and other objects is to measure changes in capacitance or resistance. Such methods have been used previously to quantify feeding behaviour in immobilized aphids [18] , [19] and larger insects [20] , but advances in digital electronics now permit this approach to be modified in a way that is compatible with greater temporal resolution, higher throughput and freely behaving animals, thereby leveraging the advantages of a genetic model organisms. We have developed an automated, high-resolution behavioural monitoring system called flyPAD (fly Proboscis and Activity Detector), that uses capacitive-based measurements to detect the physical interaction of individual Drosophila with food. To validate the accuracy of the flyPAD system, we adapted bioluminescent techniques to measure the intake of very small amounts of food as well as the dynamics of food absorption in single flies. We show that feeding from a non-liquid food induces a pattern of highly stereotyped rhythmic proboscis extensions and retractions that is suggestive of an underlying central pattern generator (CPG) controlling the feeding motor programme. The analysis of ingestion dynamics and the microstructure of meals allowed us to dissect the behavioural elements mediating the homeostatic response of the fly to starvation and satiation. These results uncover several similarities with rodents and humans, highlighting a potential conservation of strategies that regulate food intake across phyla. Hardware overview To overcome the challenge of reliably detecting and measuring physical interactions of Drosophila with substrates such as food, we developed a method based on capacitive proximity sensors. Such sensors are based on the principle of measuring the capacitance across two electrodes. We designed a sensor so that an animal standing on one electrode (electrode 1) would be in close proximity to food placed on the other electrode (electrode 2; Fig. 1a ). Whenever a fly touches the food with its proboscis or leg, it alters the dielectric constant between the two electrodes creating a change in capacitance that is large enough to be detected. We designed our system using the AD7150 (Analog Devices) ultra-low power capacitance-to-digital converter. This device allows two-channel recording at 100 Hz with a sensitivity of 1 fF. To make the measurement system compact, reproducible and scalable, we designed a printed circuit board (PCB) containing the capacitance-to-digital converter and a connector that carries the digitized capacitance signal via an I 2 C interface ( Fig. 1b ). Both the arena enclosing the fly as well as a lid were fabricated from acrylic sheets using a laser cutter and fixed on the PCB. The result is a modular arena equipped with two touch sensors, permitting experiments using a single fly with two different food sources. To allow for high-throughput recordings, we implemented an I 2 C multiplexing board on a Field Programmable Gate Array (FPGA). The resulting system can simultaneously acquire the data from 32 independent behavioural arenas and stream the data to a computer via USB interface ( Fig. 1c ). Multiple systems can be connected to a single computer, further increasing the throughput of the system. 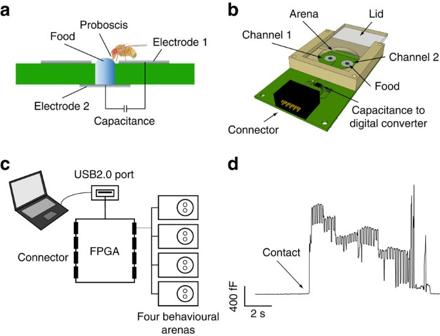Figure 1: The flyPAD setup. (a) Concept for the use of capacitance measurement to monitor the interaction of a fly with food. The interaction between the proboscis of a fly and the food is detected as a change in capacitance between two electrodes: electrode 1 on which the fly stands and electrode 2, on which the food is placed. (b) Diagram of a behavioural arena, consisting of a PCB containing the fly arena with two independent channels allowing the monitoring of feeding from two different food sources, a capacitance-to-digital converter and a connector. (c) Schematic of the complete system. Up to 32 individual behavioural arenas can be connected to an FPGA-based multiplexing board, which collects the signals and sends them to a computer via a USB interface. (d) A representative capacitance trace depicting the low level of background noise in the absence of touch and a strong change in capacitance on contact of the fly with food (as observed using a simultaneous video recording) (arrow). Figure 1: The flyPAD setup. ( a ) Concept for the use of capacitance measurement to monitor the interaction of a fly with food. The interaction between the proboscis of a fly and the food is detected as a change in capacitance between two electrodes: electrode 1 on which the fly stands and electrode 2, on which the food is placed. ( b ) Diagram of a behavioural arena, consisting of a PCB containing the fly arena with two independent channels allowing the monitoring of feeding from two different food sources, a capacitance-to-digital converter and a connector. ( c ) Schematic of the complete system. Up to 32 individual behavioural arenas can be connected to an FPGA-based multiplexing board, which collects the signals and sends them to a computer via a USB interface. ( d ) A representative capacitance trace depicting the low level of background noise in the absence of touch and a strong change in capacitance on contact of the fly with food (as observed using a simultaneous video recording) (arrow). Full size image To ground truth, the electrical signals from our device, we simultaneously monitored the behaviour of flies in the arena using a digital video camera in a series of preliminary experiments (for an example, see Supplementary Video 1 ). The contact of the fly with the food elicited an immediate increase in the capacitance signal, several orders of magnitude above the background noise of the sensor ( Fig. 1d ). The signal displayed multiple features such as rhythmic changes that appeared to be related to the interaction of the fly with the food. Automatic annotation of feeding behaviour Direct comparisons with videos suggested that whenever a fly came into contact with the food we could detect rapid changes in the amplitude of the signal for as long as the fly was active ( Figs 1d and 2a , top graph). To extract these periods of activity, we calculated the root mean square (RMS) of the signal in consecutive 500 ms windows ( Fig. 2a , middle graph). By simply thresholding this signal, it was possible to reliably extract the bouts of activity, during which the fly was interacting with the food ( Fig. 2a , grey shading in bottom graph). 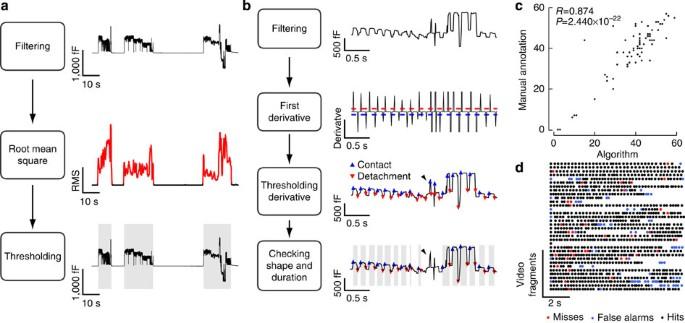Figure 2: Motor pattern extraction algorithms and validation. (a) Activity detection algorithm. Raw capacitance signal (top graph) is filtered and a RMS of the signal is calculated in a 500-ms sliding window (middle graph). Activity bouts are defined as epochs of the RMS which surpass a user-defined threshold (in red in middle graph). Extracted active food interaction bouts (activity bouts) are shaded in grey on the raw capacitance signal (lower graph). (b) Feeding detection algorithm. Capacitance trace (top graph) is filtered and differentiated (second graph from top). Positive and negative thresholds (red and blue dashed lines) are then applied to extract positive and negative deflections of the derivative. Time points of the signal where the derivative crosses the threshold are marked by blue and red arrowheads in third graph from top, indicating candidate time points for contact and detachment of proboscis with the food, respectively. The candidate contact and detachment events are assigned to form paired events based on their relative distance and size (lower graph). Black arrowhead highlights events with different shapes not corresponding to proboscis contacts with the food, which are removed by the algorithm. Segments highlighted in grey represent detected sips. (c) Validation of the feeding detection algorithm. Each dot represents the relationship between the number of proboscis contacts with food detected manually in a 10-s video fragment and the number of sips detected by the algorithm.R=Pearson Rho. (d) Validation of the temporal reliability of the sips detected by the algorithm. Each horizontal line is a 10-s period of a simultaneous capacitance and video recording. Black circles represent the coincidence of the sips detected by the algorithm and the manual annotation, red circles mark sips detected only by manual annotation and blue circles mark sips detected only by the algorithm. Figure 2: Motor pattern extraction algorithms and validation. ( a ) Activity detection algorithm. Raw capacitance signal (top graph) is filtered and a RMS of the signal is calculated in a 500-ms sliding window (middle graph). Activity bouts are defined as epochs of the RMS which surpass a user-defined threshold (in red in middle graph). Extracted active food interaction bouts (activity bouts) are shaded in grey on the raw capacitance signal (lower graph). ( b ) Feeding detection algorithm. Capacitance trace (top graph) is filtered and differentiated (second graph from top). Positive and negative thresholds (red and blue dashed lines) are then applied to extract positive and negative deflections of the derivative. Time points of the signal where the derivative crosses the threshold are marked by blue and red arrowheads in third graph from top, indicating candidate time points for contact and detachment of proboscis with the food, respectively. The candidate contact and detachment events are assigned to form paired events based on their relative distance and size (lower graph). Black arrowhead highlights events with different shapes not corresponding to proboscis contacts with the food, which are removed by the algorithm. Segments highlighted in grey represent detected sips. ( c ) Validation of the feeding detection algorithm. Each dot represents the relationship between the number of proboscis contacts with food detected manually in a 10-s video fragment and the number of sips detected by the algorithm. R =Pearson Rho. ( d ) Validation of the temporal reliability of the sips detected by the algorithm. Each horizontal line is a 10-s period of a simultaneous capacitance and video recording. Black circles represent the coincidence of the sips detected by the algorithm and the manual annotation, red circles mark sips detected only by manual annotation and blue circles mark sips detected only by the algorithm. Full size image Furthermore, on closer inspection of the videos, we noticed that flies rhythmically extended and retracted their proboscis on the food. This behaviour was reflected in a highly rhythmic, square wave-like pattern in the capacitance signal ( Figs 1d and 2b and Supplementary Video 1 ). On the basis of the hypothesis that this motor pattern might correspond to rhythmic feeding, we designed an algorithm to extract putative ‘sips’ based on the shape of the signal ( Fig. 2b , for further details see Methods). The algorithm identifies the exact moments when a sip begins (contact of the proboscis with the food) and ends (detachment of the proboscis from the food), as well as inter-sip intervals (ISIs; Fig. 2b , lower graph). To validate the accuracy of our feeding detection algorithm, we captured and manually annotated high-resolution videos from flies interacting with the food on the capacitance sensor. The number of proboscis contacts detected by manual annotation was significantly correlated with the number of sips detected by our algorithm ( Fig. 2c ). A comparison of the ethograms generated by manual annotation with the results of our automated method further confirmed the accuracy of our approach. The algorithm detected 92.5% of the sips tabulated via manual scoring, while missing 7.5% and generating 7.5% false sips ( Fig. 2d ). These data demonstrate that our method for detecting sips is sufficiently accurate to be used for automatic monitoring of feeding behaviour. Sips mediate food ingestion Although our method can reliably detect individual proboscis interactions with food (sips), it may not accurately report the actual volume that flies consume, because some proboscis extension events might represent non-ingestive sampling of the food. To test whether the automatically detected sips were correlated with actual ingestion, we developed a method for monitoring food intake in individual flies while they fed on the flyPAD. Because existing methods do not have the sensitivity required to measure food intake in real time in individual flies [4] , we exploited the capacity of the firefly enzyme luciferase to emit photons (bioluminescence) on its reconstitution with its cofactor D -luciferin [21] . It has been previously demonstrated that D -luciferin can be fed to flies and is subsequently absorbed by the nervous system [22] . Thus, photon counts generated by neuronally expressed luciferase should be temporally correlated with the intake of food mixed with D -luciferin ( Fig. 3a ). 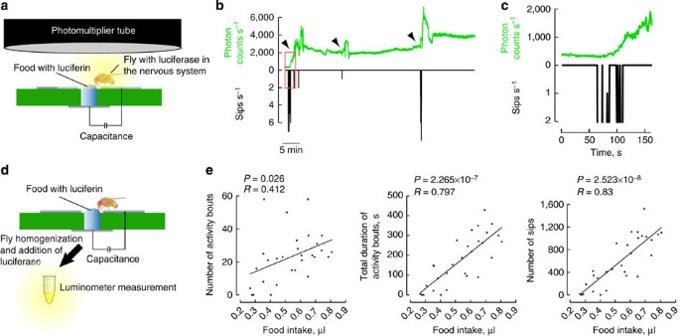Figure 3: Sips strongly correlate with food intake. (a) Schematic of the experimental setup used to measure the dynamics of food intake and the kinetics of nutrient absorption. A fly expressing luciferase in the nervous system is placed on a flyPAD with a photo multiplier tube located above to simultaneously monitor its feeding behaviour and emitted photons. The fly feeds from a 10% sucrose solution containing 10 mM luciferin. (b) Representative capacitance recording depicted as feeding rate (downward-pointing black trace) and simultaneous photon counts (upward-pointing green trace). Note that every bout of feeding leads to an increase in the photon count (arrowheads) indicating that sips lead to food ingestion and subsequent contact of luciferin with the nervous system. (c) An expanded version of the initial 160 s of the recording segment inside the orange box inb. The increase in photon counts is detected tens of seconds after the initiation of feeding, suggesting that the ingested substance reaches the nervous system quickly. (d) A schematic description of the experiment used to measure the volume of consumed food in individual flies. Feeding of flies from a food solution containing luciferin is monitored using the flyPAD. Flies are subsequently homogenized and recombinant luciferase is added to the homogenate, followed by 20 s of measurement in a 96-well plate luminometer. (e) Graphs plotting the relationship between measured food intake and the number of activity bouts (left), total duration of activity bouts (middle) and the number of sips (right).R=Pearson Rho, black line represents the regression line,n=29. Figure 3: Sips strongly correlate with food intake. ( a ) Schematic of the experimental setup used to measure the dynamics of food intake and the kinetics of nutrient absorption. A fly expressing luciferase in the nervous system is placed on a flyPAD with a photo multiplier tube located above to simultaneously monitor its feeding behaviour and emitted photons. The fly feeds from a 10% sucrose solution containing 10 mM luciferin. ( b ) Representative capacitance recording depicted as feeding rate (downward-pointing black trace) and simultaneous photon counts (upward-pointing green trace). Note that every bout of feeding leads to an increase in the photon count (arrowheads) indicating that sips lead to food ingestion and subsequent contact of luciferin with the nervous system. ( c ) An expanded version of the initial 160 s of the recording segment inside the orange box in b . The increase in photon counts is detected tens of seconds after the initiation of feeding, suggesting that the ingested substance reaches the nervous system quickly. ( d ) A schematic description of the experiment used to measure the volume of consumed food in individual flies. Feeding of flies from a food solution containing luciferin is monitored using the flyPAD. Flies are subsequently homogenized and recombinant luciferase is added to the homogenate, followed by 20 s of measurement in a 96-well plate luminometer. ( e ) Graphs plotting the relationship between measured food intake and the number of activity bouts (left), total duration of activity bouts (middle) and the number of sips (right). R =Pearson Rho, black line represents the regression line, n =29. Full size image To be able to detect photons in intact flies, we used the strong pan-neuronal Gal4 line nSyb-Gal4 to drive high levels of luciferase expression in the nervous system. On each bout of sips, we observed an increase in photon counts suggestive of food intake ( Fig. 3b,c ). Furthermore, we observed that the photon count starts increasing as quickly as 10–20 s after the first sip ( Fig. 3c ). This short delay might underlie the brief latencies previously reported for the action of metabolically active sugars in flies in appetitive conditioning [23] as well as classic flight studies [24] . This method, therefore, offers new opportunities for measuring the dynamics of nutrient absorption and nutrient availability in various tissues or cell types in the fly. Despite the advantages provided by this luciferase method, we found it difficult to quantify the exact volume of food consumed by the fly during each sip. Hence, we developed an additional assay to measure small volumes of food ingested by single flies feeding on the flyPAD. In this protocol, single flies are allowed to feed in the flyPAD from food containing D -luciferin. After the flyPAD measurement, flies are homogenized and, on addition of recombinant luciferase, the amount of light emitted is measured using a luminometer ( Fig. 3d ). The advantages of this method are that it does not require the use of luciferase-expressing transgenic animals and that the high signal-to-noise ratio of the bioluminescent signal permits the detection of very small quantities of ingested food. Comparing three different features of the capacitive signal extracted using the flyPAD (number of activity bouts, total duration of activity bouts, and number of sips) with the measured food intake allowed us to define the extent to which they correlate ( Fig. 3e ). All three behavioural metrics were correlated with ingestion; however, the degree of correlation varied. Whereas the number of activity bouts, which represent how often an animal approaches the food ( Fig. 2a ), has a significant but weak correlation with the ingested volume ( Fig. 3e , left graph), the total duration of all activity bouts ( Fig. 3e , middle graph) correlates much more strongly with food intake, as does the number of sips ( Fig. 3e , right graph). The sensitivity of this method allowed us to estimate the median volume of food that flies consume per sip to be 1.05 nl (0.72 to 1.35, 95% confidence interval). These results validate the use of the flyPAD to extract the dynamics of feeding and food intake in single flies. To demonstrate the potential applications of the flyPAD device, we next provide several examples of its use to analyse food choice, feeding motor programs and nutritional homeostasis. flyPAD allows the study of the dynamics of food choice The ability of flies to choose among foods of different qualities underlies nutrient balancing [2] and is an important experimental paradigm for uncovering the molecular and neuronal basis of gustation in Drosophila [10] , [25] , [26] , [27] . When given the choice between 1 and 5 mM sucrose in the flyPAD arena, flies strongly preferred to feed from the 5 mM sucrose source ( Fig. 4a ), as had been observed previously using the colour assay [25] . The ability to calculate the preference index for individual flies ( Fig. 4a , right side) permits the use of clonal genetic manipulations to study food choice [28] . Another parameter that strongly affects the throughput of behavioural assays is the length of each trial. Standard food choice assays are normally performed over 2 h (ref. 2 ). The cumulative plot of the preference index shows that after 10 min, the preference index plateaus at the level observed at the end of a 50 min assay ( Fig. 4b ). This suggests that using flyPAD makes it possible to drastically shorten the trial length required to make meaningful measurement of food preference. In addition, the dynamic readout of feeding provided by flyPAD permits investigation of the behavioural mechanisms underlying feeding decisions. In the case of the high- versus low-sucrose paradigm, flies continued visiting the food with the lower sucrose concentration, as visualized by a steady increase in the sip count ( Fig. 4c ). This indicates that flies did not focus exclusively on one resource, but rather continued to sample from both. The flyPAD is therefore well suited to study food choice, opening new possibilities for studying feeding decisions at a mechanistic level in Drosophila . 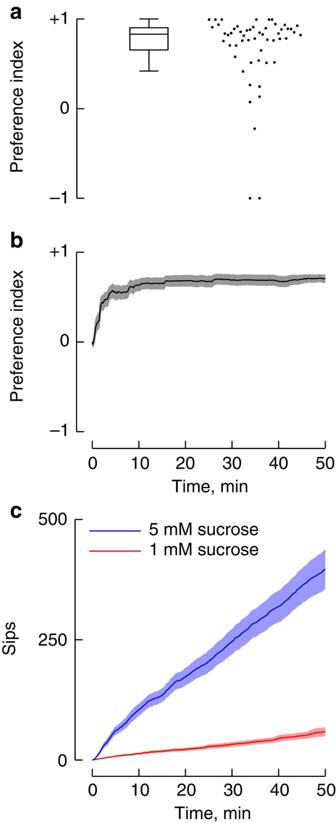Figure 4: Using flyPAD to study food choice. (a) Preference indices of flies choosing between a 1- and a 5-mM sucrose food source. Box plot displays the median, interquartile range and 5–95 percentile whiskers. Each dot in the scatter plot represents the preference index of a single fly. (b) Cumulative plot of the preference index over time. Black line represents the mean and the grey shading the s.e.m. (c) Cumulative feeding from the two different food sources over time. Line represents the mean and the shading the s.e.m.,n=55. Figure 4: Using flyPAD to study food choice. ( a ) Preference indices of flies choosing between a 1- and a 5-mM sucrose food source. Box plot displays the median, interquartile range and 5–95 percentile whiskers. Each dot in the scatter plot represents the preference index of a single fly. ( b ) Cumulative plot of the preference index over time. Black line represents the mean and the grey shading the s.e.m. ( c ) Cumulative feeding from the two different food sources over time. Line represents the mean and the shading the s.e.m., n =55. Full size image Feeding is mediated by a stable, rhythmic motor programme In humans and rodents, motor programmes underlying food ingestion such as licking, mastication and swallowing are highly rhythmic and are controlled by CPGs located in the brainstem [29] , [30] , [31] . The high temporal resolution of our system allowed us to closely analyse the structure of feeding motor patterns in flies. Similar to rodents and humans, feeding flies exhibited a highly rhythmic motor pattern, with most sips having a length of 0.13 s and an ISI of 0.08 s when eating yeast ( Fig. 5a,b ). We then tested whether either the pattern or durations of sips were modulated by the content of the food or by the internal metabolic state of the animal. We starved flies for different periods of time (0, 4 and 8 h) and then tested them on the flyPAD with a 10% sucrose gel. The durations of sips were slightly, but significantly, longer on sucrose when compared with yeast (0.16 versus 0.13 s, P =0.019, Wilcoxon Rank-Sum test) ( Fig. 5a,c ). Furthermore, the sip durations on sucrose were more variable than on yeast as evidenced by the broader distribution of the histogram. ISIs, however, were not significantly altered by the content of the food (0.07 versus 0.08 s, P =0.18, Wilcoxon Rank-Sum test) ( Fig. 5b,d ). 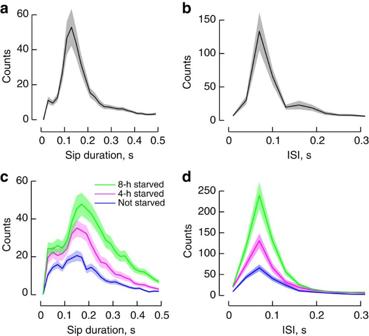Figure 5: Rhythmic feeding motor programme. (a) Distribution of the durations of sips on yeast food. (b) Distribution of ISIs on yeast food. (c) Distribution of sip durations on sucrose in three different starvation states. (d) Distribution of ISIs on sucrose in three different starvation states. All histograms are plotted with the means as solid lines and the s.e.m. as shading,n=24 for all panels. Figure 5: Rhythmic feeding motor programme. ( a ) Distribution of the durations of sips on yeast food. ( b ) Distribution of ISIs on yeast food. ( c ) Distribution of sip durations on sucrose in three different starvation states. ( d ) Distribution of ISIs on sucrose in three different starvation states. All histograms are plotted with the means as solid lines and the s.e.m. as shading, n =24 for all panels. Full size image Animals homeostatically compensate for a lack of energy by increasing their food intake following starvation. However, flies might alter their feeding motor programme in two basic ways to increase food consumption: they could increase the duration of sips (corresponding to an increase in food intake per sip) or shorten the ISIs (corresponding to an increase in the feeding rate or vigour of eating). Similar to licks in rodents [32] , we found that flies maintain both the duration of sips ( Fig. 5c ) and the ISIs ( Fig. 5d ) constant on deprivation ( P =0.078 for sip duration and P =0.35 for ISI, Kruskal–Wallis one way analysis of variance). Therefore, the feeding motor programme of Drosophila consists of a highly rhythmic proboscis extension and retraction cycle suggestive of an underlying CPG. This pattern is not altered substantially by changes in the internal hunger state of the animal, but does partially adapt to the nature of the food. The microstructure of feeding reveals homeostatic strategies If the motor programme underlying feeding is not modified following starvation, how does a hungry fly modify feeding to achieve homeostasis? In rodents, meals are organized in ‘bursts’ of licking [13] , and an increase in feeding following starvation is achieved mainly by reducing the interval between bursts [33] , [34] . To dissect the behavioural strategies leading to increases in food intake following starvation in Drosophila, we analysed changes in the microstructure of meals. On the basis of criteria established for rat licking behaviour [13] , we defined a feeding burst as three or more consecutive sips separated by inter-burst intervals (IBIs) smaller than double the median ISI ( Fig. 6a ). In fully fed flies, sips were organized into bursts consisting of an average of 5.8 sips ( Fig. 6b ). Whereas the length of the feeding bursts was not significantly altered after 4 h of starvation, 8 h of starvation led to a significant increase in the number of sips per feeding burst (average of 8.3 sips). In contrast to feeding bursts, just 4 h of starvation led to a significant shortening of the IBI from 78 to 29 s ( Fig. 6c ). Additional starvation (8 h) did not cause a further decrease in IBI. The dissociable effects of starvation time on the duration of feeding bursts and IBI suggest that flies use distinct strategies to adapt to short and medium lengths of starvation. After a short period of starvation, the fly is active on the food for longer periods ( Fig. 6d ) and shortens the intervals between feeding bursts ( Fig. 6c ). On longer starvation times, the fly also increases the length of the feeding bursts ( Fig. 6b,k ). 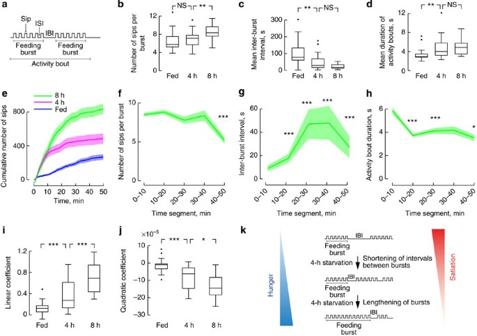Figure 6: Feeding behaviour microstructure reveals homeostatic strategies. (a) Illustration of the temporal dynamics of feeding of a fly on gelatinous food and of the different parameters measured and analyzed using the flyPAD approach. (b) Mean number of sips per burst, (c) mean IBI length and (d) mean duration of activity bouts in fully fed, 4 h starved and 8 h starved animals. (e) Cumulative feeding for the same three groups. Line represents the mean and the shading the s.e.m. (f) Number of sips per burst, (g) duration of the IBI and (h) duration of activity bouts for five consecutive 10-min time windows over the course of a meal. Inf–h, lines represent the mean and the shading the s.e.m.; significance was tested compared with the first window. (i) Linear and (j) quadratic coefficients extracted from quadratic fit to the cumulative feeding of individual flies (Supplementary Fig. 1) in fully fed, 4- and 8-h starved conditions. (k) Model of how hunger and satiation induce stepwise changes in feeding strategies to achieve homeostasis. Box plots display the median, interquartile range and 5–95 percentile whiskers, with data beyond these whiskers shown as points. NS, not significant (P>0.5), *P≤0.05, **P≤0.01, ***P≤0.001, Significance was tested by Wilcoxon Rank-Sum test with Bonferroni correction,n=24. Figure 6: Feeding behaviour microstructure reveals homeostatic strategies. ( a ) Illustration of the temporal dynamics of feeding of a fly on gelatinous food and of the different parameters measured and analyzed using the flyPAD approach. ( b ) Mean number of sips per burst, ( c ) mean IBI length and ( d ) mean duration of activity bouts in fully fed, 4 h starved and 8 h starved animals. ( e ) Cumulative feeding for the same three groups. Line represents the mean and the shading the s.e.m. ( f ) Number of sips per burst, ( g ) duration of the IBI and ( h ) duration of activity bouts for five consecutive 10-min time windows over the course of a meal. In f – h , lines represent the mean and the shading the s.e.m. ; significance was tested compared with the first window. ( i ) Linear and ( j ) quadratic coefficients extracted from quadratic fit to the cumulative feeding of individual flies ( Supplementary Fig. 1 ) in fully fed, 4- and 8-h starved conditions. ( k ) Model of how hunger and satiation induce stepwise changes in feeding strategies to achieve homeostasis. Box plots display the median, interquartile range and 5–95 percentile whiskers, with data beyond these whiskers shown as points. NS, not significant ( P >0.5), * P ≤0.05, ** P ≤0.01, *** P ≤0.001, Significance was tested by Wilcoxon Rank-Sum test with Bonferroni correction, n =24. Full size image Whereas hunger increases food intake to compensate for the lack of nutrients, satiation regulates the length of a meal by inducing its termination. The effect of satiation is reflected in the reduction of the slope in the cumulative number of sips ( Fig. 6e ). To quantify how the three microstructure parameters change as the animal becomes satiated, we calculated how each changed during a meal ( Fig. 6f–h ). We performed these calculations for the flies starved for 8 h, because the satiation effect is the strongest ( Fig. 6e ). As expected, over the duration of the meal all parameters reverted to values approximating the situation in fully fed flies. The number of sips per burst only significantly changed at the end of the meal, from 8.5 sips per burst at the beginning to 5.2 sips per burst at the end of the experiment ( Fig. 6f ). A significant change in the length of the IBI and the duration of activity bouts is already detected within about 10 min after the start of a trial ( Fig. 6g,h ). The modulation of these feeding parameters during the meal ultimately leads to its termination ( Fig. 6e ). The initial rate of feeding can be used as a bona fide measurement of the motivation to feed. The deceleration of food intake, on the other hand, can be used as readout for the strength of the satiation signal leading to the termination of a meal [14] , [35] . Satiation is difficult to measure in Drosophila , so we used an approach employed in human feeding research and fitted a quadratic equation [35] to the cumulative feeding curves of every individual fly and extracted the linear and the quadratic coefficients from the fitted curves ( Supplementary Fig. 1 ). As expected, the linear coefficients (which in vertebrates is a proxy for the motivation to feed) increases following starvation ( Fig. 6i ) [14] . Likewise, the quadratic coefficient (which is thought to represent the strength of the satiation signal) decreases significantly following starvation ( Fig. 6j ) [14] . These results indicate that in flies, as in humans, the linear and the quadratic coefficients are good readouts for the drive-to-eat and the satiation signals. We use a new device based on capacitive sensing to study the interaction of Drosophila melanogaster with food. This has allowed us to study feeding behaviour at a temporal resolution of 100 samples per second and with <nl sensitivity in individual flies. Our design allows the flies direct access to the food in an unrestricted way, eliminating possible confounds created by the use of capillaries. Although flyPAD is very sensitive, it is easy to implement and operate and automatically generates critical feeding metrics related to total food intake, hunger and satiation. The technology provides a powerful method for studying feeding phenotypes related to nutritional homeostasis [1] , [2] , aging [36] , diabetes [37] , [38] and obesity [38] , [39] . The technology should also lend itself to study other types of behaviour in which a fly interacts with a substrate, such as egg laying [40] , [41] , by correlating behavioural features with the capacitance signal. Monitoring feeding over the whole life time of flies would be valuable for specific fields such as aging. While the current version of the flyPAD does not lend itself to this timescale, it should be possible to adapt it in the future. One possibility would be to use liquid food that could be stored in containers that automatically refill the wells. By combining the flyPAD approach with tissue-specific bioluminescence, we were able to estimate the timescale from the intake of a substance to its incorporation within the nervous system. The fact that D -luciferin is an amphipathic molecule at physiological pH and that it therefore relies on active transport to enter tissues, makes it a suitable proxy to monitor nutrient uptake [42] , [43] . Interestingly, the timescale we measured is on the order of 10–20 s. Our direct measurements support the notion that the nervous system of flies has very fast access to the nutrient content in food, and that the animal can use this post-ingestive information to control behaviour [23] . Using cell-specific drivers, one should be able to measure the timescale of nutrient availability in different tissues including individual classes of neurons. The latter experiments should be able to clarify whether nutrient-sensitive neurons in Drosophila [6] , [7] have privileged access to the nutrient content of food, as it is the case in vertebrates [44] . The high temporal resolution of our method allowed us to identify motor patterns as well as behavioural strategies used by the fly to homeostatically control food intake. Feeding in flies consists of a sequence of proboscis extensions and retractions [8] , [45] . We show that this motor pattern is rhythmic and is likely controlled by a CPG. A pair of interneurons was recently described to control the initiation of the feeding programme in Drosophila [8] . It is conceivable that these neurons could be connected to the CPG network, a hypothesis that could be tested in future studies. We have found that the frequency of the motor rhythm is affected by the physical properties of the food. This result is in agreement with earlier findings in other insects that the CPGs controlling chewing are modulated by sensory feedback [46] , [47] . We measured the proboscis extension and retraction cycle and found that, similar to the motor programme controlling pumping of liquid foods, the pattern is not modified by the internal state of the animal but can be altered by the content of the food [48] . Despite this similarity, the motor programs for feeding from liquid and gelatinous food differ in an important way. When a fly ingests a liquid, its proboscis remains in contact with the food for sustained pumping [48] , whereas feeding on gelatinous food involves an additional motor behaviour consisting of rhythmic extensions and retractions of the proboscis. This more complex motor programme for gelatinous food could have evolved to either deposit salivary gland extracts, to mechanically scrape off ingestible quantities of food, or to support the local probing of the nutrient content on heterogeneous substances such as fruits. The microstructure of feeding behaviour has been used in different organisms to obtain mechanistic insights into the behavioural underpinnings of homeostasis [12] , [13] , [14] , [15] . More precise, time-resolved measures of behaviour permit the differentiation of specific aspects of feeding regulation such as the drive to initiate and terminate a meal [12] , [33] . We have shown that Drosophil a organizes sips into feeding bursts that cluster together to form a meal. On a short period of starvation (4 h), the spacing between bursts shortens significantly. On longer starvation periods (8 h), the burst length increases leading to a progressive increase in the total number of sips and therefore an increase in food intake. This increase in burst length is anticipated by an increase in the time a fly interacts with the food after 4 h of starvation. Therefore, flies appear to deploy different behavioural strategies to compensate for the lack of food in a hierarchical sequence rather than a graded fashion. It is important to note that by the end of the feeding assay, the total number of sips was not significantly different between fully fed and 4-h starved animals, suggesting that these two groups cannot be differentiated by considering only total feeding. Satiation seems to act inversely on these feeding parameters, reverting them to values similar to the fully fed situation and thus leading to termination of the meal. In flies, dopamine has been shown to mediate the effect of starvation on gustatory sensitivity [49] , [50] ; however, the effect of longer starvation periods on the gustatory neurons does not seem to depend on this neuromodulatory pathway [49] . These data suggest that the fly might use separate molecular and behavioural mechanisms to control homeostasis of food intake depending on the severity of the hunger state. Approaches allowing detailed characterization of feeding and further improvements in behavioural analysis such as unbiased segmentation of behaviour into bouts [51] , [52] will aid in obtaining a more complete picture of the mechanisms underlying homeostasis. The molecular mechanisms controlling metabolism and physiology in Drosophila appear to be largely conserved with other organisms [38] . However, it is not clear whether the behavioural strategies controlling food intake are conserved to the same extent across phyla. We show that several features of feeding behaviour in flies appear to be similar to the ones described in vertebrates. The proboscis extension and retraction cycle in flies and licking in rodents are rhythmic motor patterns that are neither modulated by the sensory properties of the food nor the internal state of the animal [32] . Furthermore, licking in rodents [13] and the proboscis extension cycle in flies are organized in bursts and one of the key parameters modulated by hunger is the spacing between these bursts [33] . Finally, the regulation of the cumulative intake curve by the internal state of the animal also appears to be similar in flies, rodents and humans [14] . The aforementioned parallels between the different animal models suggest that the organization of motor patterns regulating food intake and their homeostatic control share striking similarities across phyla. Our work opens up new avenues for studying the neuronal basis of feeding behaviour and food intake at different time scales in an automated and high-throughput manner. The ability to subdivide homeostatic changes in feeding into specific changes in feeding strategies opens up new opportunities to explore how molecular mechanisms, neuronal circuits and metabolic processes interact to control food intake and nutrient homeostasis to optimize life history traits such as reproduction and aging. Fly stocks and rearing conditions w 1118 flies were used for all experiments except for the real-time bioluminescence experiments. For the real-time bioluminescence experiments, a third chromosomal nSyb-Gal4 (generated by Julie Simpson) strain was used to drive the expression of a UAS-luciferase transgene (generated by Georg Dietzl and Barry J. Dickson). Flies were reared at 25 °C, 60% humidity using a 12-h light–dark cycle. The medium contained, per liter, 80 g cane molasses, 22 g beetroot syrup, 8 g agar, 80 g corn flour, 10 g soya flour, 18 g yeast extract, 8 ml propionic acid and 12 ml nipagin (15% in ethanol). Behavioural experiments For yeast feeding experiments, 5–7-day old female flies were wet starved for 12 h. Flies were then transferred into a behavioural arena by mouth aspiration and left to feed on a 10% yeast solution (SAF instant yeast) in 1% agarose. For the choice experiments, 5–7-day old male flies were wet starved for 24 h before testing. Flies were then transferred into a behavioural arena by mouth aspiration and allowed to choose between 1 mM sucrose and 5 mM sucrose solutions dissolved in 1% agarose. For the experiments testing the effect of starvation on sucrose feeding, 5–7-day old male flies were wet starved for 0, 4 and 8 h, respectively, before testing. Flies were then transferred into a behavioural arena by mouth aspiration and left to feed on a 10% sucrose solution dissolved in 1% agarose. All the food solutions used in the experiments were prepared by dissolving 1% agarose at 70 °C in a water bath, adding the relative nutrient, dividing the solution into 2 ml aliquots and freezing them at −20 °C. For each experiment, the aliquots were melted again at 70 °C in a heat block immediately before the experiment. For some experiments, each arena was placed into a small Faraday cage made of aluminium foil and connected to the ground of the power supply to remove potential noise. Hardware design, FPGA code and data acquisition PCBs were designed in Eagle CAD software (CadSoft). The PCB production was done by Eurocircuits ( http://www.eurocircuits.com/ ). Fly arenas were designed in Inkscape ( www.inkscape.org ) and cut on a laser cutter (Epilog) from transparent 3 mm acrylic. FPGA code was written in VHDL using Quartus 2 web edition software (Altera Corporation). The feeding sensor uses the principle of capacitive proximity sensing, and is based on the AD7150 integrated circuit, with a resolution of 1.0 fF. There are two electrodes per sensor, the outer ‘fly’ electrode 1 and the inner ‘food’ electrode 2. The electrode assembly is constructed as a two-sided PCB, where the outer electrode is a foil trace and the inner electrode is a through-plated via. The outer electrode consists of an annular trace with an outer diameter of 10 mm and an inner diameter of 3 mm. The inner electrode has a diameter of 1.75 mm, and is accessed using a trace on the bottom side of the PCB. The AD7150 uses two sense signals per channel, an excitation output and a capacitive input. The excitation output connects to the outer electrode, and the capacitance input connects to the inner electrode. Each integrated circuit contains two sensing channels. We use both to monitor two neighbouring feeding sensors per chip in each arena. To increase experimental throughput, thirty-two dual-channel behavioural arenas are connected via I 2 C serial interface to a multiplexer based on the Altera Cyclone IV EP4CE22F17C6N FPGA (as part of a Terasic DE0-Nano board). The multiplexer communicates with each AD7150 in a round-robin fashion, and makes the readings available through a FTDI serial USB interface. To acquire the streamed capacitance data, we developed a package for the Bonsai data stream processing framework [53] (available at https://bitbucket.org/horizongir/bonsai.neuro ). We also used Bonsai to simultaneously acquire data from video capture devices. For all the analyses, we used a capacitance signal acquired at 100 Hz. All subsequent signal processing and data analysis steps were done in Matlab (Mathworks). Hardware designs and software are available at http://www.flypad.pt . Activity bout detection To remove slow fluctuations in capacitance that are likely to occur in some cases due to subtle changes in food distribution on the electrodes caused by fly feeding as well as by the evaporation of food from the electrode, we detrended the signal by subtracting the low-passed version of the signal from the original capacitive trace. The low-passed version of the signal was obtained by convolving the signal with a 500-ms square wave. The resulting trace kept all the fine features of the original trace but did not drift over time and had a mean of zero. To estimate when the fly was actively exploring/eating the food, we calculated the RMS of the signal in consecutive 500 ms windows ( Fig. 2a , middle panel). The high signal-to-noise ratio and low variability of the background signal allowed us to use a fixed threshold of 10 RMS units for all our traces to select epochs of increased fly activity. Activity bouts were defined as epochs of the RMS that surpassed the threshold. To compensate for the delay introduced by the windowed RMS calculation, we subtracted 400 ms from the beginning and the end of each of the activity bouts. For each of the activity bout, we extracted a set of parameters which were later used in the analysis, namely the time of the initiation and the termination of the sip, sip duration and ISI. Sip detection The signal was processed the same way as for the activity bout detection. To detect putative sips, we differentiated the signal ( Fig. 2b , second panel from the top). The derivative revealed periodic positive and negative peaks. To extract these peaks, we calculated a positive threshold and a negative threshold separately using the method proposed by Rodrigo Quian Quiroga [54] for unbiased detection of action potentials. Positive and negative thresholds ( T ) were calculated as follows: Where σ is an estimate of the s.d. of the noise and x are all non-zero positive and negative values of the derivative of the signal. To account for the non-stationary nature of the signal we divided the data into 3-s intervals and calculated the thresholds separately for each of them. Positive values of derivative that exceeded the positive threshold were considered putative attachments of the proboscis and the negative values exceeding the negative threshold were considered as putative detachments of the proboscis. Out of these putative events, we further selected only the local absolute maxima within 70 ms. To remove the events with a shape different from the square wave, we assigned putative attachments and detachments of the proboscis to pairs and removed the events with a duration shorter than 40 ms and longer than 3 s as well as events with amplitude of the detachment signal with a value less than 50% of the attachment ( Fig. 2b , arrowheads in bottom panel). Validation of the sip detection algorithm and food intake We placed a flyPAD behavioural arena under a SteREO Discovery.V12 (Carl Zeiss) stereo microscope equipped with a Flea 3 (Point grey) USB 3.0 camera. Flies were allowed to feed on yeast in the flyPAD while being recorded on video at 50 f.p.s. The synchronization between the flyPAD capacitance signal and the video was implemented in Bonsai. Only video segments in which all the proboscis contacts could be seen (no obstructions by other body parts of the fly) were included in the analysis. Selected videos were annotated by inspecting the videos frame by frame and manually annotating the time of contact of the proboscis with the food. To compare the performance of the algorithm with the manual annotation we compared both the extracted timepoint of attachment of the proboscis to the food and the number of proboscis extensions (sips) in 10 s video segments. To validate food intake, we used a real-time bioluminescence method: a photo multiplier tube (H7360-02, Hamamatsu) was placed immediately above the flyPAD behavioural arena and connected to a photon counting unit (C8855-01, Hamamatsu). The whole setup was placed in a light tight environment. Female flies expressing luciferase in their nervous system were left to feed in a behavioural arena containing luciferin-laced food prepared by mixing 10% sucrose with 10 mM firefly D -luciferin Na+ salt ( D -luciferin sodium salt ref L3708 from Melford Biolaboratories) in 1% agarose [55] . To validate the food intake, we also used a volumetric bioluminescence method: the luciferase-containing food was prepared the same way as described in the section above, except that we used 10% yeast instead of 10% sucrose. Flies were allowed to feed on the flyPAD for 1 h. Immediately afterwards, flies were individually collected from the flyPAD and homogenized in 50 μl 1 × Glo Lysis buffer (Promega), briefly spinned using a table top centrifuge (to remove air bubbles), resuspended and 20 μl of the resulting solution was added to 100μl of QuantiLum Recombinant Luciferase diluted in 900 μl 1X Glo Lysis buffer. The photon counts were measured twice for 20 s per well in a 96-well plate using a MicroLumat Plus LB96V microplate reader (Berthold Technologies). The average of the two reads was used for further analysis. The calibration curve was generated by serially diluting luciferase-containing food. The resulting data points were fit to a power law function ( R 2 =0.997) and the resulting equation was used to translate the photon counts into the consumed volume of food. To avoid a distortion by the dark counts produced by the photomultiplier, data points that corresponded to less than 20 sips were not used for the calculation of the ingested volume per sip. Data analysis Preference index ( Fig. 4a ) was calculated as follows: PI=( n 5− n 1)/( n 5+ n 1), where n 1 and n 5 are the number of sips on 1 and 5 mM sucrose, respectively. The cumulative preference index plot ( Fig. 4b ) was calculated using the same formula where n 1 and n 5 are the number of sips at consecutive 10 s moments in time ( Fig. 4c ). Motor behaviours (sip durations and inter-sip intervals) were analysed by calculating the histogram for each individual fly using 30 ms bins. For the comparison of motor patterns across different conditions, we used the modes (corresponding to the peak in the histogram) of the sip duration and the ISI. Feeding bursts were defined as three or more consecutive sips with an ISI of less than two median ISIs of each fly. Cumulative number of sips was calculated in 10 s bins. How to cite this article: Itskov, P. M. et al. Automated monitoring and quantitative analysis of feeding behaviour in Drosophila . Nat. Commun. 5:4560 doi: 10.1038/ncomms5560 (2014).